Low-concentration mechanical biosensor based on a photonic crystal nanowire array The challenge for new biosensors is to achieve detection of biomolecules at low concentrations, which is useful for early-stage disease detection. Nanomechanical biosensors are promising in medical diagnostic applications. For nanomechanical biosensing at low concentrations, a sufficient resonator device surface area is necessary for molecules to bind to. Here we present a low-concentration (500 aM sensitivity) DNA sensor, which uses a novel nanomechanical resonator with ordered vertical nanowire arrays on top of a Si/SiO 2 bilayer thin membrane. The high sensitivity is achieved by the strongly enhanced total surface area-to-volume ratio of the resonator (10 8 m −1 ) and the state-of-the-art mass-per-area resolution (1.8×10 −12 kg m −2 ). Moreover, the nanowire array forms a photonic crystal that shows strong light trapping and absorption over broad-band optical wavelengths, enabling high-efficiency broad-band opto-thermo-mechanical remote device actuation and biosensing on a chip. This method represents a mass-based platform technology that can sense molecules at low concentrations. Nanoelectromechanical systems [1] , [2] are enabling emerging applications in biosensing [3] , [4] , [5] , [6] , [7] , [8] , [9] , [10] , [11] , due to their extraordinary sensitivities in mass changes. For mass-change-based nanomechanical biosensors, there are two important metrics [12] . The first one is its minimum detectable mass, which is defined as its absolute mass sensitivity. The resonance frequency of a nanoelectromechanical systems resonator is a sensitive function of its total mass. By measuring the resonance frequency change of the resonator, the mass change could be detected. Achieving small detectable mass changes requires the resonator to be light and operated at a high-quality factor [13] . The second metric is the minimum detectable mass per area, which is named as mass-per-area sensitivity and defined to be the minimum detectable mass divided by the surface sensing area of the device [12] . The mass-per-area sensitivity is useful for comparing concentration sensitivity. When a biosenor is immersed into a target solution at a certain concentration, the total mass of the biomolecules bound to the sensor surface will be proportional to its surface sensing area, at fixed time in the linear region. For nanomechanical biosensing [14] at low concentrations, it requires not only minimum detectable mass but also large device surface area for molecules to bind to. Nanomechanical cantilevers showed single-molecule level absolute mass sensitivity [4] , [12] , [15] , [16] , [17] and the single DNA molecule was detected [17] . However, single DNA detection [17] requires high concentrations of DNA solution (10 −9 mol l −1 ) to get even a single DNA binding, due to the small surface area of the device. A recent report [14] , indicated that the challenge for new biosensors is to achieve low limits of concentration detection. Therefore, achieving high concentration sensitivity of a biosensor leads to a requirement of a minimum device detectable mass per area, instead of a minimum detectable mass only. Here we present a novel nanomechanical resonator device with ordered vertical nanowire (NW) arrays on top of a Si/SiO 2 bilayer thin membrane. The device shows strongly enhanced total surface area-to-volume ratio 10 8 m −1 and the state-of-the-art mass-per-area resolution 1.8×10 −12 kg m −2 , enabling biomolecule sensing in low-concentration target solution. As an example, a label-free DNA sensor is demonstrated, showing 500 aM concentration sensitivity. Compared with previous reported label-free mechanical mass-based sensing techniques [5] , [7] , [8] , [9] , [10] , [14] our NW array biosensor shows the state-of-the-art concentration sensitivity. Moreover, the NW array forms a photonic crystal that shows strong light trapping and absorption over broad-band optical wavelengths, enabling high-efficiency opto-thermo-mechanical actuation of the resonator. The optical energy coupling directly into the device eliminates the need for any interconnect wires, and could enable high-efficiency remote optically driven actuation and biosensing on a chip. Device structure and fabrication The surface area-to-volume ratio of our ordered NW array resonator is extremely large (up to 10 8 m −1 ). This is nearly two and three orders of magnitude larger than that of the micro-cantilever [17] and the suspended microchannel resonators [6] , [12] , respectively. This large surface area-to-volume ratio allows highly effective surface-based biomolecular mass sensing, especially at low target concentrations ( Fig. 1 ). For device fabrication, electron beam lithography was used to pattern SiO 2 nano-post arrays on a silicon-on-insulator (SOI) wafer. Si NW arrays were created by silicon reactive ion etching (RIE), using patterned SiO 2 nano-posts as the etching mask. Optical lithography was used to pattern the backside circular cavity, using backside alignment. Silicon deep RIE was used to etch through the silicon substrate using the SOI-buried oxide as the stopping layer. 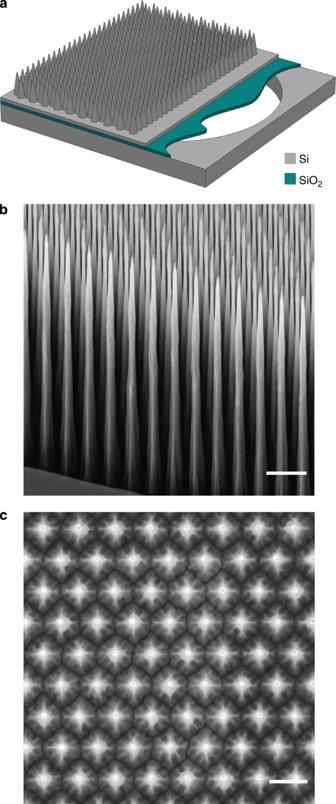Figure 1: Device structure of the photonic crystal NW arrays mechanical resonator. (a) Schematic representation of device structure, with ordered vertical Si NW arrays on top of the Si/SiO2(300 nm/200 nm) membrane. The outer surface of NWs on membrane region was coated with a thin Ti/Au (2 nm/3 nm) passivation layer (not shown here). (b) SEM image (40° side view) of the Si NW arrays, with 1.7 μm wire height, 100 nm wire base diameter, ~5 nm tip, at a 100 nm pitch. (c) SEM image (top view) of the NW arrays inb. The scale bars inbandcare 200 nm and 100 nm, respectively. Figure 1: Device structure of the photonic crystal NW arrays mechanical resonator. ( a ) Schematic representation of device structure, with ordered vertical Si NW arrays on top of the Si/SiO 2 (300 nm/200 nm) membrane. The outer surface of NWs on membrane region was coated with a thin Ti/Au (2 nm/3 nm) passivation layer (not shown here). ( b ) SEM image (40° side view) of the Si NW arrays, with 1.7 μm wire height, 100 nm wire base diameter, ~5 nm tip, at a 100 nm pitch. ( c ) SEM image (top view) of the NW arrays in b . The scale bars in b and c are 200 nm and 100 nm, respectively. Full size image Enhanced broad band light absorption for NW arrays The photonic crystal NW arrays presented highly anti-reflective optical properties (black surface, Fig. 2a ). Light incident onto the NW arrays can be absorbed and converted to heat efficiently via photon absorption. This was confirmed by the infrared camera image ( Fig. 2b ), showing that the NW area temperature increased much faster than that for the surrounding planar Si area, when they are irradiated by a white light lamp. In the measured light absorption spectra curves ( Fig. 2c ), the NW array shows strongly enhanced light trapping and absorption efficiency, over a broad-band wavelength of 400–900 nm, as compared with that for the planar control Si thin film. This is consistent with previous predictions and reports [18] , [19] , [20] . 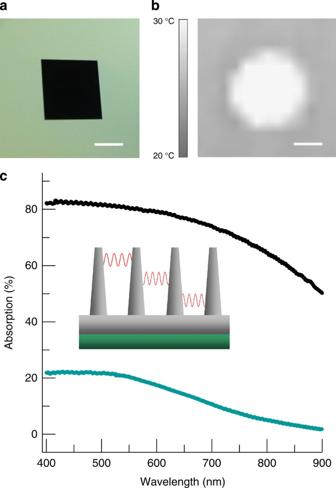Figure 2: Enhanced broad-band light absorption measurements for the photonic crystal NW arrays. (a) Photograph image of device top surface with NW arrays (black area). (b) Infrared camera image of the NW sample, irradiated by a white light lamp (10 mW) in air. The NW area (white) was heated up much faster than the surrounding planar Si area (grey). It might be due to the heat diffusion that the hotter area is not well square shaped as the initial shape ina. The scale bars inaandbare both 500 μm. (c) Measured light absorption spectra of the membrane (300 nm Si) with NW on top (black curve), compared with that of bare planar thin Si membrane (2 μm thick, cyan curve). For both samples, the surfaces have the same thin passivation layer Ti/Au (2 nm/3 nm). Inset shows the schematic illumination of the enhanced light trapping mechanisms for photonic crystal Si NW arrays. Figure 2: Enhanced broad-band light absorption measurements for the photonic crystal NW arrays. ( a ) Photograph image of device top surface with NW arrays (black area). ( b ) Infrared camera image of the NW sample, irradiated by a white light lamp (10 mW) in air. The NW area (white) was heated up much faster than the surrounding planar Si area (grey). It might be due to the heat diffusion that the hotter area is not well square shaped as the initial shape in a . The scale bars in a and b are both 500 μm. ( c ) Measured light absorption spectra of the membrane (300 nm Si) with NW on top (black curve), compared with that of bare planar thin Si membrane (2 μm thick, cyan curve). For both samples, the surfaces have the same thin passivation layer Ti/Au (2 nm/3 nm). Inset shows the schematic illumination of the enhanced light trapping mechanisms for photonic crystal Si NW arrays. Full size image High-efficiency opto-thermo-mechanical device actuation The strong broad-band light trapping and absorption optical properties of the photonic crystal NW arrays enable the high-efficiency opto-thermo-mechanical excitation for the resonator. An intensity modulated laser light ( λ =680 nm) was focused onto the membrane ( Fig. 3a ). The heating from the incident modulated light leads to bending moments in the Si/SiO 2 laminate ( Fig. 3b ), due to the differences in the coefficient of linear thermal expansion in the two layers. This opto-thermo-mechanical actuation takes advantage of direct coupling of optical energy into selected device areas, eliminating the electrical interconnects required in integrated electrostatic or piezoelectric actuation and enabling high-efficiency remote optically driven actuation for biosensing. Compared with previous planar Si nano-mechanical resonator actuation methods by local laser heating [21] , [22] , our excitation technique has the following advantages. First, the excitation efficiency of the photonic crystal NW array resonator has an enhancement factor of 5 to 30 over the measured spectral range 400–900 nm, compared with the control planar Si thin film resonator ( Supplementary Methods and Supplementary Fig. S1 ). Second, the wavelength of our driving light can be broadband, ranging from ultraviolet to near infrared. In biosensing, this broad-band excitation capability enables the protection of the biomolecules that are sensitive to high-energy photons [23] , by using low-energy photon excitation, such as near infrared range. 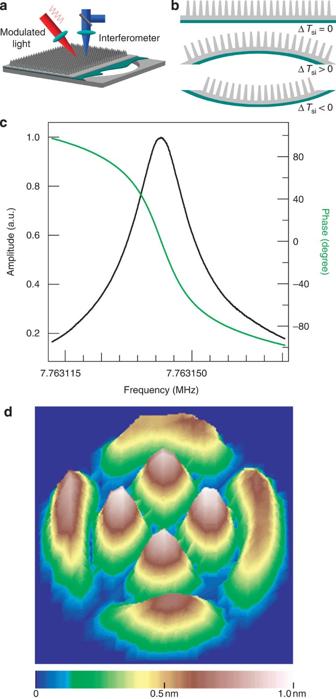Figure 3: Opto-thermo-mechanical actuation for the photonic crystal NW array mechanical resonator and its response. (a) Schematic representation for the experiment setup. Intensity-modulated light was used to actuate the membrane resonator and the vibration responses were measured using PolyTec interferometer with phase-locked loop. (b) Schematic for Si/SiO2-bending moments induced by the local heating from the modulated laser, due to the thermal expansion coefficient differences between the bilayer materials. The periodic temperature difference (ΔTSi) necessary for device excitation is expected to be <0.1 °C. (c) Measured amplitude and phase of the resonator's response showing a mode resonance at 7.76314 MHz. This mode has a high quality factor up to Q~3.2×105. The resonator consists of vertical NW arrays on Si/SiO2bilayer membrane, with membrane diameter of 50 μm. (d) Measured standing-wave vibration amplitude 2D mapping pattern of the mode inc. During mapping, the optical actuation frequency was fixed at the resonance mode and the interferometer laser gun was controlled by a stage controller for lateral movement with sub 0.5 μm lateral resolution. Figure 3: Opto-thermo-mechanical actuation for the photonic crystal NW array mechanical resonator and its response. ( a ) Schematic representation for the experiment setup. Intensity-modulated light was used to actuate the membrane resonator and the vibration responses were measured using PolyTec interferometer with phase-locked loop. ( b ) Schematic for Si/SiO 2 -bending moments induced by the local heating from the modulated laser, due to the thermal expansion coefficient differences between the bilayer materials. The periodic temperature difference ( ΔT Si ) necessary for device excitation is expected to be <0.1 °C. ( c ) Measured amplitude and phase of the resonator's response showing a mode resonance at 7.76314 MHz. This mode has a high quality factor up to Q~3.2×10 5 . The resonator consists of vertical NW arrays on Si/SiO 2 bilayer membrane, with membrane diameter of 50 μm. ( d ) Measured standing-wave vibration amplitude 2D mapping pattern of the mode in c . During mapping, the optical actuation frequency was fixed at the resonance mode and the interferometer laser gun was controlled by a stage controller for lateral movement with sub 0.5 μm lateral resolution. Full size image The thermo-optically excited vibration response of the laminate was measured using a PolyTec interferometer ( Fig. 3a ) with a phase-locked loop, which has a resolution of <0.1 nm in vibration amplitude resolution. One of the mechanical modes possesses highest quality factor up to 3.2×10 5 , as shown by the frequency response plot in Figure 3c . The high quality factor of the resonator (in vacuum 0.1 mTorr) might be due to the reduced surface loss [24] and clamping loss [25] , through proper Si surface high-temperature annealing treatment processes and the induced tensile stress to the Si film, respectively ( Supplementary Discussion ). Measured standing-wave vibration amplitude 2D mapping pattern of this mode was shown in Figure 3d . During mapping, the optical actuation frequency was fixed at the resonance mode and the interferometer laser gun was controlled by a stage controller for lateral movement with sub 0.5 μm lateral resolution. The measured standing-wave pattern of this mode matched well with the simulated mode pattern of the circular membrane ( Supplementary Fig. S2 ). The NW array resonator detection scheme relies on the resonance frequency shift due to the mass change after biomolecule attachment. The resonance frequency, f , could be expressed as: with resonator spring constant k , effective mass m eff , mass change δm and a numerical constant α that depends on the geometric localization of the added mass ( Supplementary Methods ). Based on equation (1), when m eff > δm , the resonance frequency shift, δf , could be expressed as: where f 0 is the initial resonant frequency of the resonator. Device mass responsivity was measured by adding various known mass to the sensor, through chemisorption of thiolated single-stranded DNA molecules ( Supplementary Methods and Supplementary Fig. S3 ). The measured mass responsivity is (9.0±0.4) Hz fg −1 . With the experimentally determined frequency uncertainty of 1 Hz, the measured minimum absolute mass resolution of our resonator is 1.1×10 −19 kg. Using the measured total surface area 6.1×10 −8 m 2 of the resonator, the measured mass-per-area sensitivity is determined to be 1.8×10 −12 kg m −2 , which is around two and four orders of magnitude larger than that for the previous suspended micro-channel resonator [12] and micro-cantilever resonator [17] , respectively ( Table 1 ). Our photonic crystal NW array resonator shows the state-of-the-art mass-per-area sensitivity, compared with other reported mechanical mass biosensors. Table 1 Sensitivity comparison with other mechanical mass sensors. Full size table Low-concentration DNA sensor demonstration With high mass-per-area sensitivity, the resonator enables high-sensitivity surface-based detection of biomolecules at ultra-low concentrations. This is proved by demonstrating a low-concentration DNA sensor. For DNA detection, single-stranded probe DNA molecules with known sequence are immobilized onto the gold-coated NW surface and followed by surface passivation with mercaptohexanol [26] ( Fig. 4a ). Although the planar gold surface is hydrophilic (52° contact angle), the gold-coated NW array structure is superhydrophilic (8°, Supplementary Fig. S4 ), which is good for solution-based biomolecule detection. 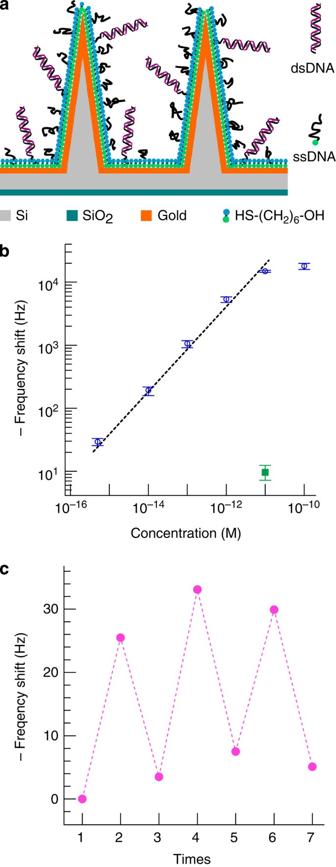Figure 4: Low-concentration DNA detection. (a) Schematic representation of the DNA immobilization and hybridization. (b) Measured resonance frequency shift, plotted as a function of target concentration. The dashed fitting line is also added. The control experiment, using 10 pM non-matching DNA, is shown by a green square. The error bars present s.e. values on the mean, for multiple measurements (n=3). The frequency shows saturation at concentrations above 10 pM. (c) Measured sensor responses for repeated DNA hybridization at 500 aM target solution and dehybridization. The resonance frequency shows negative shift (29.3±2.5 Hz) after DNA hybridization (even times) and resonance frequency shift goes to background noise level (5.4±2.0 Hz) after DNA dehybridization (odd times except the first time). Figure 4: Low-concentration DNA detection. ( a ) Schematic representation of the DNA immobilization and hybridization. ( b ) Measured resonance frequency shift, plotted as a function of target concentration. The dashed fitting line is also added. The control experiment, using 10 pM non-matching DNA, is shown by a green square. The error bars present s.e. values on the mean, for multiple measurements ( n =3). The frequency shows saturation at concentrations above 10 pM. ( c ) Measured sensor responses for repeated DNA hybridization at 500 aM target solution and dehybridization. The resonance frequency shows negative shift (29.3±2.5 Hz) after DNA hybridization (even times) and resonance frequency shift goes to background noise level (5.4±2.0 Hz) after DNA dehybridization (odd times except the first time). Full size image For DNA hybridization, we carried out the control experiment against a non-matching DNA sequence at 10 pM concentration first and then the hybridization experiments for matching sequence at varying target DNA concentrations from 500 aM up to 10 pM. The resonance frequency negative shift has a well-defined linear relation with the target DNA concentration ( Fig. 4b ). The demonstrated concentration sensitivity (500 aM) of our DNA sensor represents enhancement of one to six orders of magnitude in the detection limit, compared with the previously reported label-free DNA detection methods [17] , [27] , [28] , [29] . The reusability of our device is also demonstrated ( Fig. 4c ). The resonance frequency shows negative shift (29.3±2.5 Hz) after DNA hybridization at 500 aM target solution and the shift goes to background noise level (5.4±2.0 Hz) after DNA dehybridization. Similar reusability demonstration was also shown with high concentration 10 pM target solution in Supplementary Figure S5 . Compared with the non-reusable device of previous multi-step chemical-amplified DNA detection techniques, the reusability of our device can potentially greatly reduce the cost. In addition, cost can be further reduced by using our recently reported technique, high-throughput self-powered parallel electron lithography [30] , [31] , to pattern the NW arrays, instead of using the expensive and low-throughput electron beam lithography. The mass-per-area sensitivity of mechanical resonators is critical for solution concentration detection [12] . Biosensing at low concentrations using mechanical resonators requires not only low detectable mass but also a large device surface area for molecules to bind to. Although the absolute mass sensitivity of our NW array resonator does not advance the state-of-the-art value, our sensor achieves the highest mass-per-area sensitivity among all the nanomechanical biosensors ever reported, to our best knowledge. This high mass-per-area sensitivity of our sensor enables biomolecule detection at low concentrations. As an example, a reusable low-concentration DNA sensor has been realized using this photonic crystal NW array mechanical resonator. It shows 500 aM concentration sensitivity. Compared with previously reported label-free mass-based mechanical biosensing techniques, our NW array biosensor shows the state-of-the-art low concentration sensitivity [3] , [5] , [7] , [8] , [9] , [14] . A recently reported atomic force microscopy approach [32] showed attomolar DNA concentration resolution by label-free imaging of single hybridized DNA molecules, based on the stiffness differences between single- and double-stranded DNA molecules. Compared with that, our method eliminates the requirement for direct contact with the molecules that might cause sample damage. Moreover, our device provides a potential way for the low-concentration detection of biomolecules that are not suitable for stiffness-change-based probing. Moreover, the strongly enhanced light trapping and optical absorption from the photonic crystal NW arrays enables high efficiency opto-thermal-mechanical actuation of the resonator over broad-band optical wavelengths. It takes advantage of coupling optical energy directly into the device efficiently, eliminating any additional interconnect electrical wires and enabling remote optically driven actuation and biosensing on a chip. In biosensing, this broad-band excitation capability enables the protection of the biomolecules that are sensitive to high-energy photons, by using low-energy photon excitation, such as near-infrared range. Another important advantage of our photonic crystal NW array mechanical-resonator detection technique is that it is compatible with multiplexed analysis using microarray platforms. High-resolution lithographic techniques are used for device fabrication and that can create a large number of nearly identical sensing elements on the same chip, which integrates well with systems. The high-efficiency optical actuation and detection approach enables the rapid interrogation of array elements, allowing for multiplexed analysis. Photonic crystal NW array resonator fabrication Dry SiO 2 (100 nm) was formed on the top surface of a SOI wafer (Si (2 μm)/SiO 2 (0. 2 μm)/Si (200 μm) stack) at 1,000 °C. A thick layer of plasma-enhanced chemical vapor deposition (PECVD) SiO 2 (3 μm, at 400 °C) was deposited on the backside of the SOI wafer. A thin layer of negative tone chemical-amplified e-beam resist NEB31A was spun on top of the dry SiO 2 surface, followed by electron beam lithography (100 keV beam energy) patterning and normal NEB31A development process. Ordered SiO 2 post arrays were formed by silicon dioxide RIE, using NEB31A as the etching mask. Si NW arrays were created by Si RIE (70 sccm of BCl 3 , 2 sccm of H 2 , 20 mTorr), using SiO 2 posts array as the etching mask. The Si NW height could be controlled by etching time and 300 nm of planar Si under the NW arrays remained after etching. Then the sample was annealed at 1,000 °C for 30 s in vacuum, to remove the organic absorber on the Si surface and the crystal defects caused by previous Si RIE. A thin layer of Ti/Au (2 nm/3 nm) was deposited to passivate the outer surface of the NW, by the conformal CHA evaporator at low deposition rate. In the deposition process, the surface area enhancement factor by the NW structure needs to be considered. Then the top side was coated with a thick layer of photoresist stack (LOR (~1 μm)/SPR 220-4.5(~5 μm)) to protect the NW arrays for following backside processes. Circular cavity was formed on the backside PECVD SiO 2 layer, using EV620 contact aligner photolithography with backside alignment and followed the SiO 2 RIE process. A layer of SiO 2 (1 μm) was patterned to cover the whole chip top surface except the circular membrane region, with optical photolithography patterning, SiO 2 deposition and lift off. This SiO 2 layer was used to cover the Au surface that will not be used for DNA detection. Finally, a membrane was formed by etching through the SOI wafer Si substrate, using Si deep reactive ion etching (SF 6 ) with the PECVD back oxide as the mask and the buried oxide as an etch stop. Optical absorption spectra measurement Both reflectance ( R ) spectra and transmittance ( T ) spectra measurements were conducted, using a xenon lamp combined with a monochromator. The absorption ( A ) spectra was calculated by A =100%− R − T . A small part of diffusely reflected light was not included in the reflection measurements, due to the experimental setup limitations. Therefore, the absorption spectra represent an upper limit. Opto-thermo-mechanical device actuation Modulated laser light (680 nm wavelength) was used to actuate the membrane resonator in vacuum (0.1 mTorr). The vibration responses were measured using PolyTec interferometer with phase-locked loop, which has a resolution of <0.1 nm in vibration amplitude. During standing-wave vibration amplitude 2D mapping ( Fig. 3d ), the optical actuation frequency was fixed at the resonance mode and the interferometer laser gun was controlled by a stage controller for lateral movement with sub 0.5 μm lateral resolution. Based on the measured standing-wave 2D mapping pattern, the mode can be determined. Therefore, we can make sure that the shifted mode comes from the same initial vibration mode. DNA immobilization and hybridization Thiolated single-strand DNA (1 μM, IDT) was tethered to the freshly prepared gold surface in 1.0 M KH 2 PO 4 buffer (PH=4.1). Immobilization was carried out at room temperature for 3 h, followed by copious rinsing with distilled water (18.2 MΩ cm). Mercaptohexanol (1 mM) was then used to remove nonspecific binding and passivate the gold surface for 1 h. DNA hybridization was carried out in 1 ml of the hybridization buffer (1.0 M NaCl with TE buffer (10 mM Tris and 1 mM EDTA, pH=8.2)) at 37 °C for 2 h under constant mixing. After hybridization, the device was rinsed with TE buffer to remove nonspecific DNA bindings, followed by volatile salt ammonium acetate solution (10 mM) rinsing and dried in a weak stream of nitrogen. The volatile salt can be removed in vacuum within several minutes. Control experiment was carried out in 10 pM non-matching DNA in hybridization buffer. For DNA dehybridization, the device was soaked in 55 °C TE buffer three times, 10 min each. Then the device was rinsed with distilled water and dried in nitrogen. DNA sequences Probe DNA for immobilization: 5′-CACGACGTTGTAAAACGACGGCCAG-3′ Target DNA: 5′-CTGGCCGTCGTTTTACAACGTCGTG-3′ Control non-matching DNA: 5′-TCGCGCATCAATGCTGATACTAGTC-3′ How to cite this article: Lu, Y. et al . Low-concentration mechanical biosensor based on a photonic crystal nanowire array. Nat. Commun. 2:578 doi: 10.1038/ncomms1587 (2011).